Controlling the symmetry of inorganic ionic nanofilms with optical chirality Manipulating symmetry environments of metal ions to control functional properties is a fundamental concept of chemistry. For example, lattice strain enables control of symmetry in solids through a change in the nuclear positions surrounding a metal centre. Light–matter interactions can also induce strain but providing dynamic symmetry control is restricted to specific materials under intense laser illumination. Here, we show how effective chemical symmetry can be tuned by creating a symmetry-breaking rotational bulk polarisation in the electronic charge distribution surrounding a metal centre, which we term a meta-crystal field. The effect arises from an interface-mediated transfer of optical spin from a chiral light beam to produce an electronic torque that replicates the effect of strain created by high pressures. Since the phenomenon does not rely on a physical rearrangement of nuclear positions, material constraints are lifted, thus providing a generic and fully reversible method of manipulating effective symmetry in solids. The symmetry environment of metal centres in compounds defines many of their functional properties. Dynamic control of material symmetry consequently allows time varying switching of properties required for device applications [1] . Lattice strain is the most natural agent for tuning symmetry properties since it physically alters the relative positions of constituent chemical species. Light–matter interactions have been used to provide a controllable means of introducing strain into certain materials. They can induce strains that would otherwise require extreme external forces, and they can enable states of matter to be reached that are inaccessible with adiabatic thermodynamic processes [2] , [3] . However, a fundamental weakness of using such light–matter interactions is that they are non-generic, relying on a material-specific property, such as the presence of either a phase transition [2] , [3] , [4] , [5] , [6] or weakly bound layers [7] in crystalline solids. This greatly limits the range of materials that can be optically tuned and hence restricts potential applications. Circularly polarised light (CPL) can induce symmetry reduction in chemical environments of photoactive materials [8] , [9] , [10] , [11] , an ability that is associated with its inherent sense of handedness, a property known as chirality, conveyed by its intrinsic spin angular momentum. Effectively the inherent sense of twist of the spin angular momentum of the CPL is transferred to the physical structure, breaking mirror symmetry. However, conventionally CPL can only act as a symmetry-reducing influence in photoactive systems, which either have a chiral component or have the potential to be chiral. There has been no previous evidence that illuminating an intrinsically non-chiral photo-inactive material with CPL can alter the symmetry properties of the chemical environments of the constituent species. In contrast to atomic dimensions, transfer of optical spin angular momentum can impart a sense of physical twist on a much longer length scale. Angular momentum transfer from CPL has been used in opto-mechanics to impart torques to rotate mesoscale objects about the incident beam axis [12] , [13] , [14] , [15] . However, the torques are far too weak to break chemical symmetry by physically distorting chemical bonds. Consequently, the potential of chiral light for symmetry breaking in materials that have no chiral character has never been established. Here we demonstrate a chiral light–matter effect for reversibly manipulating the effective symmetry of chemical environments within a solid material, without requiring a physical distortion of the chemical structure. We propose that the effect arises from a transfer of optical spin angular momentum from a chiral light beam through an interfacial mechanism. The mechanism involves the transfer of optical spin angular momentum to create an “electronic torque” that distorts the electron density surrounding a metal centre. The resulting bulk polarisation, which circulates around the incident beam, acts as a symmetry-reducing perturbation on the local chemical environment. By analogy with the crystal field established by ligands around a coordinated metal ion, the bulk polarisation effectively acts as a “meta-crystal field” to create an electrostatic potential that acts as a second-order perturbation on the symmetry environment of the metal centres. This effect is considered to be generic for ionic inorganic films containing transition and lanthanide metal ion centres. Here, we establish the efficacy of the phenomenon using 150-nm-thick Eu 2 O 3 nanofilms deposited on a transparent polycarbonate substrate. Eu 2 O 3 films were chosen because Eu 3+ is exquisitely sensitive to its co-ordination environment and the symmetry-reducing effects of the meta-crystal field can be detected in-situ using luminescence spectroscopy. The sole role of the Eu 3+ is that of a spectator probe ion and it is not specifically necessary for the creation of the meta-crystal field. In a second experiment, we use chiral nanostructures to modulate the amount of spin angular momentum transferred to the Eu 2 O 3 films. In both cases, symmetry reduction is reversible because the electronic torque is removed when the light is switched off. Experimental results are complemented with numerical finite-element simulations allowing the spin transfer to be quantified directly, demonstrating this effect as the cause of changes in Eu 3+ luminescence owing to symmetry reduction. Continuity equation for optical chirality Angular momentum endows light with a handedness which for our purposes can conveniently be quantified by the optical chirality density, C [16] , [17] , [18] , [19] : 
    C = 1/2( 𝐃·𝐁̇ - 𝐁·𝐃̇),
 (1) where D is the displacement field, B the magnetic induction and \({\dot{\mathbf{D}}}\) and \({\dot{\mathbf{B}}}\) are their respective time-derivatives. In free space, the optical chirality density is conserved, but interfaces act as sinks and sources of chirality. In order to derive a continuity equation for the optical chirality at an interface, we introduce a complex permittivity, \(\varepsilon = \varepsilon^\prime + i\varepsilon^{\prime\prime}\) , and permeability, \(\mu = \mu^\prime + i\mu^{\prime\prime}\) , and assume that the incident light is sufficiently narrow band that ε and μ can be approximated as being independent of frequency. The real fields in Eq. ( 1 ) are also written in terms of: \({\mathbf{D}} = ( {\varepsilon {\pmb{\cal{E}}} + \varepsilon^\ast {\pmb{\cal{E}}}^\ast } )\) and \({\mathbf{B}} = \left( {\mu {\pmb{\cal{H}}} + \mu^\ast {\pmb{\cal{H}}}^\ast } \right)\) . Differentiating Eq. ( 1 ) with respect to time yields the following narrow band continuity equation [20] (see Supplementary Note 1 ): 
    Ċ - iω∇·[ ε^'( E×E^∗) + μ^'( H×H^∗) ]_chirality flux
     	= iω ^2 ( E·H^∗ - H·E^∗) ( μ^'ε^'' + ε^'μ^'')_loss term
       + iω[ ( ∇ε^') ·( E×E^∗) + ( ∇μ^') ·( H×H^∗) ]_interface-exchange term (IE). (2) The left-hand side has the typical form for a conserved quantity with the time derivative of the chirality density and the divergence of its flux. The right-hand side includes a loss term corresponding to absorption and an interface–exchange (IE) term showing how chirality is lost or generated whenever the real part of the permittivity or permeability changes. This is in contrast to the optical helicity [21] , which is conserved when the interface preserves the duality symmetry of the free electromagnetic (EM) field [22] , [23] . For nonmagnetic or weakly magnetic systems ∇ μ ′ can be neglected. The implication of the IE term is that for CPL propagating through a transparent planar film with two inequivalent interfaces there can be a net non-dissipative transfer of chirality to the medium. Since this transfer depends on the real part of the dielectric response, it physically manifests as a polarisation within the material, which has a sense of direction about the incident beam. Specifically, the chirality flux is proportional to the spin angular momentum of the light, and its spatial change is balanced by an effective torque embodied by the interface term, which is therefore responsible for the polarisation distortion. The meta-crystal field model In the case of the Eu 2 O 3 films described here, we propose that the polarisation derives from a collective distortion of an ensemble of O 2− ions, which are more polarisable than the smaller Eu 3+ ion; this reduces the effective symmetry of the co-ordination environment of the Eu 3+ . Crystal field theory describes the lifting of the degeneracy of the electronic states of a cationic metal centre by the electrostatic field produced by its nearest-neighbour anionic co-ordination environment [24] . By analogy, the “meta-environment” of an ensemble of polarised anions creates a chiral electrostatic field that perturbs the symmetry of the metal ion. In effect, the symmetry-reducing meta-crystal field is created by an electronic torque caused by the transfer of spin angular momentum arising from the exchange of optical chirality. Our proposed electronic torque is a macroscopic phenomenon, which acts over the whole irradiated area, creating an electrostatic polarisation with a local direction that precesses through 360°, Fig. 1a . On the length scale of the Eu 3+ co-ordination environment, all the oxygen atoms would be polarised in the same direction. The induced polarisation breaks mirror symmetry, unless the incident light is orthogonal to a mirror plane of the co-ordination environment, Fig. 1b . Turning now to the data, Fig. 2a presents luminescence spectra collected from Eu 2 O 3 films under a variety of conditions. Eu 3+ luminescence spectra originate from f – f transitions ( 5 D 0 → 7 F J , where J = 1–4). The 5 D 0 → 7 F 2 emission of Eu 3+ ∼ 615 nm (subsequently denoted 7 F 2 ) is referred to as hypersensitive, being highly sensitive to the local environment of the ion compared to the other transitions [25] (see Supplementary Fig. 1 ). Luminescence spectra can consequently be used to characterise the local structure of the Eu 2 O 3 film. All of the films used show qualitatively similar luminescence spectra where the 7 F 2 is the most prominent band and they are consistent with the Eu 3+ co-ordination environment being a mixture of those found in cubic and monoclinic Eu 2 O 3 [26] . The films lack long-range order and transmission electron microscopy indicates them to be amorphous (Supplementary Fig. 2 ). Amorphous films have significant benefits for the current study: (a) they prevent the occurrence of birefringent effects that would introduce artefacts into fluorescence measurements; and (b) they illustrate that the effect is independent of crystal structure, demonstrating its generic nature. This lack of crystallinity implies that Eu 2 O 3 formula units will be randomly oriented throughout the film, but the local co-ordination and nearest-neighbour point-group symmetry about Eu 3+ ions is expected to retain the co-ordination site types found in crystalline phases: C s symmetry in monoclinic-like and C 2 and S 6 , respectively, in the cubic-like environments [27] , [28] . Previous work has shown that Eu 3+ ions with C s and C 2 symmetries in the monoclinic and cubic-like environments exhibit a 7 F 2 emission band with relatively high intensities compared to other symmetry environments [29] . Hence any reduction in local symmetry (e.g., C s → C 1 ) as a result of the meta-crystal field results in a decrease in the relative intensity of the 7 F 2 emission band. Fig. 1: Meta-crystal fields and symmetry reduction. a The graphic illustrates the precession of the induced polarisation (represented by the ellipsoids) over an extended length scale. The incident CPL is shown. For simplicity the effect is illustrated with an idealised periodic lattice, the real films are structurally disordered. b The symmetry-reducing effects of the meta-crystal field illustrated for a monoclinic-like co-ordination environment (green and blue spheres/ellipsoids are Eu 3+ and O 2− ions, respectively). A range of propagation directions relative to the mirror plane normal (dotted line) are shown. The red and green areas represent mirror planes, which have been lifted or retained, respectively, after the application of the meta-crystal field perturbation. The point group of the perturbed lattice is given beside the structure. Full size image Fig. 2: Optical chirality transfer modifies the luminescence of unstructured Eu 2 O 3 films. a The relative intensity of the hypersensitive 7 F 2 luminescence peak decreases when illuminated with CP compared to linear light if the two interfaces (air-Eu 2 O 3 and Eu 2 O 3 -polycarbonate in this case) have differential gradients. b , c The relative luminescence intensity decreases for CP light with input light power, but remains constant for LP light, owing to increasing optical chirality transfer in the former. d Numerical simulation of the change in C with distance from the input on passing through air, Eu 2 O 3 and polycarbonate, using thicknesses of 300 nm (air), 150 nm (Eu 2 O 3 ) and 350 nm (polycarbonate) for the three films. The magnitude of the IE terms for each interface is highlighted by the red arrow, and the net exchange of C , ΔIE is given. Full size image Luminescence and simulations of Eu 2 O 3 films A comparison of 7 F 2 emission spectra for unstructured films in air, excited by linearly polarised (LP) and left and right CPL (LCP and RCP) is shown in Fig. 2a . Since LP is not chiral, this spectrum is a reference for a non-perturbed Eu 3+ environment. Both LCP and RCP spectra are identical and display a reduction in the relative intensity of the 7 F 2 emission indicative of a lowering in the effective symmetry environment of Eu 3+ . The relative intensity of CPL 7 F 2 emission decreases with increasing laser power, shown in Fig. 2b , and the data fit well to a straight line with a negative gradient. A linear dependence is consistent with an increasing electronic torque, produced by a greater rate of exchange of optical spin angular momentum with increasing light intensity, creating a larger symmetry-reducing perturbation. As expected for non-chiral LP light there is no dependency of relative emission intensity with power, shown in Fig. 2c . The exchange of optical chirality would be expected to be non-linear only for high intensity laser pulses when higher order terms of the electronic permittivity become significant. Finite-element EM simulations have been performed to illustrate how C changes as CPL propagates through the films studied, which agree with Eq. ( 2 ). In these simulations, using COMSOL Multiphysics models of the substrate, Eu 2 O 3 , and analyte layers were created with additional integration surfaces (slices) added at regular intervals to allow C to be calculated with distance through the sample. The level of the symmetry-reducing perturbation is dependent only on the magnitude of the net C transferred and not its sign. Consequently, C is normalised to that of the incident polarisation, so it is always positive. From these simulations the magnitudes of the IE term in Eq. ( 2 ) can be calculated. The magnitude of the net transfer of C to a film (ΔIE) for an incident polarisation is defined as follows: 
    ΔIE = IE_inc - IE_out,
 (3) where IE inc and IE out are, respectively, the magnitudes of C exchanged at the incident and exit surfaces for the propagating light. In Fig. 2d are the numerical simulations of C for an unstructured flat Eu 2 O 3 film in air. As expected, given the refractive indices (RI) of air (RI = 1) and polycarbonate (RI = 1.619) IE inc > IE out and ΔIE = 0.05 for both LCP and RCP light. By covering the air interface with microscope oil (RI = 1.518), the RI environment becomes closer to that of the polycarbonate substrate, so that the numerical simulations, Fig. 3a , give ΔIE ≈ 0 for both CP of light. In the absence of a net exchange of chirality, Fig. 3b shows no difference between LP and CP spectra, indicating no significant symmetry-reducing perturbation. Fig. 3: Optical chirality transfer with equivalent interfaces (oil-Eu 2 O 3 -polycarbonate). a Luminescence spectra normalised to 7 F 1 for LP (black) and LH (red) and RH (blue) CPL. b The equivalent numerical simulation to that is shown in Fig. 2 d for the oil-Eu 2 O 3 - polycarbonate case, using thicknesses of 300 nm (oil), 150 nm (Eu 2 O 3 ) and 350 nm (polycarbonate) for the three films. Full size image Nanostructured Eu 2 O 3 metafilms In a second experiment, we modulated the magnitude of ΔIE using nanostructured chiral metafilms (see Supplementary Fig. 3 for images). The Eu 2 O 3 from which these films are composed is identical to that above and is amorphous and achiral on atomic length scales, so that Eu 3+ does not display any intrinsically chiral properties. Scattering CP and LP light from chiral nanostructures has previously been shown to create near fields, which exhibit spatial variations in both intensity and C (Supplementary Fig. 4 ). The values of C can locally be either greater or less than that of the incident CPL alone [30] . Consequently, the overall value of \(( \pmb{\cal{E}} \times \pmb{\cal{E}}^\ast )\) in Eq. ( 2 )—and hence the amount of C exchanged—can differ from that discussed in Figs. 2 and 3 . The level of C transferred is dependent on the exact nature of the chiral structure. The metafilms used in this study were chosen because they do not give rise to final state effects that would affect the luminescence intensities (see Supplementary Note 2 and Supplementary Fig. 5 ). It should be noted that in contrast to unstructured surfaces, scattering of LP from chiral metafilms can also generate chiral near fields [31] and thus transfer C to a film, albeit to a lesser extent than for CP light. Luminescence spectra were collected for LCP and RCP from left-handed (LH) and right-handed (RH) forms of each of the three types of chiral metafilms. To highlight the CP dependency, we present difference spectra (RCP minus LCP) for the three types of metamaterial, illustrated in Fig. 4 (see Supplementary Fig. 6 for individual spectra). As one would expect, the difference spectra collected from LH and RH structures are qualitatively equal and opposite. The signs of the difference spectra correlate with the difference in C transferred by RCP and LCP (ΔIE RCP − ΔIE LCP ). 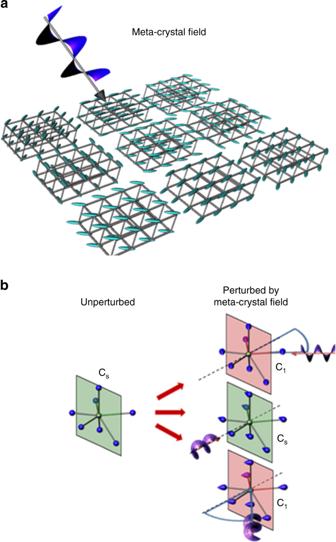Fig. 1: Meta-crystal fields and symmetry reduction. aThe graphic illustrates the precession of the induced polarisation (represented by the ellipsoids) over an extended length scale. The incident CPL is shown. For simplicity the effect is illustrated with an idealised periodic lattice, the real films are structurally disordered.bThe symmetry-reducing effects of the meta-crystal field illustrated for a monoclinic-like co-ordination environment (green and blue spheres/ellipsoids are Eu3+and O2−ions, respectively). A range of propagation directions relative to the mirror plane normal (dotted line) are shown. The red and green areas represent mirror planes, which have been lifted or retained, respectively, after the application of the meta-crystal field perturbation. The point group of the perturbed lattice is given beside the structure. A detailed method for these calculations and the associated values are given in Supplementary Note 2 and Supplementary Table 1 , respectively. A positive (negative) difference in the amount of C transferred corresponds to difference spectra with negative (positive) senses. The correlation between ΔIE RCP − ΔIE LCP and magnitude of the difference spectra is qualitative. 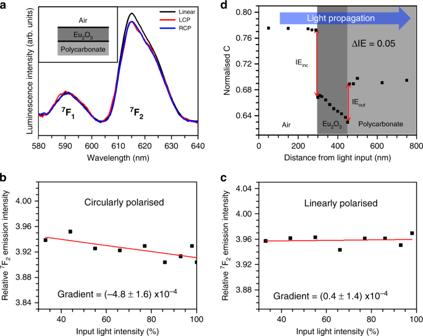Fig. 2: Optical chirality transfer modifies the luminescence of unstructured Eu2O3films. aThe relative intensity of the hypersensitive7F2luminescence peak decreases when illuminated with CP compared to linear light if the two interfaces (air-Eu2O3and Eu2O3-polycarbonate in this case) have differential gradients.b,cThe relative luminescence intensity decreases for CP light with input light power, but remains constant for LP light, owing to increasing optical chirality transfer in the former.dNumerical simulation of the change inCwith distance from the input on passing through air, Eu2O3and polycarbonate, using thicknesses of 300 nm (air), 150 nm (Eu2O3) and 350 nm (polycarbonate) for the three films. The magnitude of the IE terms for each interface is highlighted by the red arrow, and the net exchange ofC, ΔIE is given. A comparison between the asymmetry parameter, g , and the amount ΔIE RCP − ΔIE LCP is given in Supplementary Table 2 . As expected, the 500 × 500 structure, which has the largest exchange of chirality, gives the largest g . It should be stressed that the idealised structures in the EM modelling procedure do not account for defects in the real structures, which may alter the amount of optical chirality transferred. 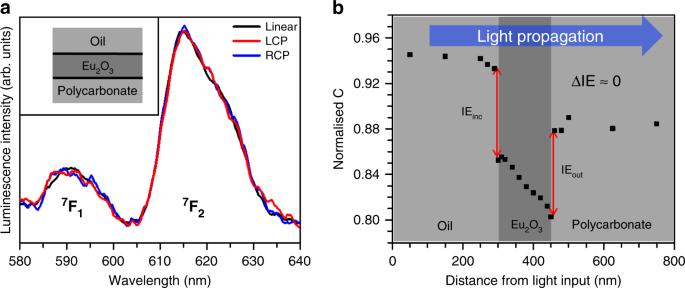Fig. 3: Optical chirality transfer with equivalent interfaces (oil-Eu2O3-polycarbonate). aLuminescence spectra normalised to7F1for LP (black) and LH (red) and RH (blue) CPL.bThe equivalent numerical simulation to that is shown in Fig.2d for the oil-Eu2O3- polycarbonate case, using thicknesses of 300 nm (oil), 150 nm (Eu2O3) and 350 nm (polycarbonate) for the three films. 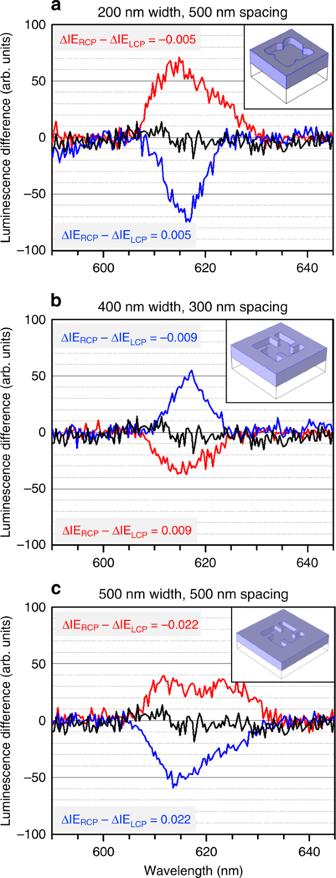Fig. 4: Luminescence difference spectra for metafilms. a,cshow the difference in luminescence RCP–LCP for the LH nanostructure (red), RH nanostructure (blue) and equivalent unstructured surface (black). The LH and RH structures show opposite differences at the7F2peak. The width and spacing labels equate to the lateral size and interstitial spacing of the nanostructures, respectively, ΔIERCP− ΔIELCPvalues for each handedness of structure are shown (red and blue for LH and RH structures, respectively), demonstrating the same equal and opposite behaviour as the difference spectra. Insets show structure geometries not drawn to scale (see Supplementary Fig.3for scale diagrams). There is no simple correlation between nanostructure geometry (i.e., width and spacing) and the amount of chirality transferred to the substrate. An absence of complete mirror symmetry within pairs of experimental difference spectra are a result of small variations in the geometries of the nanostructures that occur as a result of the fabrication process. Fig. 4: Luminescence difference spectra for metafilms. a , c show the difference in luminescence RCP–LCP for the LH nanostructure (red), RH nanostructure (blue) and equivalent unstructured surface (black). The LH and RH structures show opposite differences at the 7 F 2 peak. The width and spacing labels equate to the lateral size and interstitial spacing of the nanostructures, respectively, ΔIE RCP − ΔIE LCP values for each handedness of structure are shown (red and blue for LH and RH structures, respectively), demonstrating the same equal and opposite behaviour as the difference spectra. Insets show structure geometries not drawn to scale (see Supplementary Fig. 3 for scale diagrams). Full size image Extensive literature, since the 1960s, describes the use of Eu 3+ luminescence to probe local co-ordination environment [25] , enabling the present data to be placed into context. The changes in 7 F 2 emission observed here are equivalent to those produced by ∼ 1% compressive lattice strain in crystalline systems, produced through ion substitution [32] or the application of GPa pressures [33] . These levels of perturbation are significant and are sufficient, for example, to manipulate superconducting [34] and magnetoresistive [35] properties in other systems. Creating meta-crystal fields through the exchange of optical chirality provides a mechanism to make a broad range of materials photo-responsive. Thus, the phenomenon lifts the constraints on materials that can be exploited in opto-electronics, thus providing the opportunity for novel functionalities. Given that the phenomenon originates from an interfacial mechanism it could be an ideal candidate for the optical control of topological properties. Luminescence setup The 404 nm laser diode was driven using a 180 mA fixed current, resulting in a maximum optical power output of ~17 mW measured using a digital power meter equipped with a photodiode sensor. Luminescence spectra in Figs. 2 a, 3a and 4 were measured at this power. For power dependence measurements, shown in Fig. 2 and Supplementary Fig. 7 , 17 mW was defined as 100% output. For excitation with LP light, luminescence spectra were collected using an orthogonal polarisation, which reduced the background. The same output polarisation was used to monitor luminescence excited by CPL. See Supplementary Fig. 8 for a diagram of the setup. Polycarbonate substrate fabrication The templated substrates were made using an injection moulding machine (ENGEL), following the technique described by Gadegaard et al. [36] . The master shim for this was made using electron beam lithography. To create the master, 100 nm of poly(methyl methacrylate) resist was spin coated onto a Si wafer and baked for an hour at 180 °C. The resist is patterned using a VB6 UHR EWF lithography tool (Raith). The exposed resist was developed in IPA and methyl isobutyl ketone, MIBK (3:1 ratio) for 60 s, then rinsed in copious amounts of IPA before dried in a stream of nitrogen gas. The shim for injection moulding was prepared by electroplating from the patterned resist master. The nano patterns were indentations in the surface and had a depth of ~80 nm, range from 200 to 500 nm in length from arm to arm, and inter-structure spacing from 300 to 500 nm. When Eu 2 O 3 was deposited on the surface, it uniformly coats the substrate and takes the shape of the indentation to form a structure constituting an “inverse” hole structure at the top and a solid one at the bottom. The nanostructures have subsequently been given labels of the general form ( A × B ), where A and B are, respectively, the lateral dimensions and separations of nanostructures in nanometres. Eu 2 O 3 deposition Films were deposited by pulsed laser deposition (PLD) using sintered Eu 2 O 3 targets (Pi Kem Ltd., UK) in 50mTorr pressure of oxygen. Deposition was conducted at room temperature directly onto structured polycarbonate substrates in a Neocera Pioneer PLD vacuum system, employing a Coherent Compex Pro KrF excimer laser (248 nm, 20 ns pulses, 18 Hz, up to 200 mJ pulse energy). The target was rotated during deposition to minimise the transfer of particulates to the sample. The film structure was then characterised by transmission electron microscopy by deposition a ~40-nm-thick film directly onto an amorphous holey carbon film and imaged in a JEOL ARM CFEG instrument operated at 200 kV. Supplementary Fig. 2 presents a typical image of the edge of the film, which appears structureless. Neither a Fourier transform nor a selected area electron diffraction image (both inset to the figure) reveals sharp spots or rings that would indicate crystallinity. A single, diffuse ring is observed in diffraction that is characteristic of an amorphous, or glassy material. Numerical electromagnetic modelling EM simulations were performed using a commercial finite-element package (COMSOL v4.4, Wave optics module). Periodic boundary conditions were used to emulate the meta-film arrays. Perfectly matched layer conditions were used above and below the input and output ports. Varying polarisations of EM wave were applied at normal incidence onto the films. COMSOL uses the finite-element method to solve Maxwell’s equations over a specified geometry with fields and optical chirality being measured at pre-defined surfaces above, within, and below the films. For Eu 2 O 3 interpolation functions in terms of wavelength for the real and imaginary parts of refractive index were identified from two sources [37] , [38] and each implemented to identify a best fit compared to experimental data. Paramagnetic behaviour of the Eu 2 O 3 was accounted for by including a relative magnetic permeability of 1.01 [38] .